TRPA1 channels mediate acute neurogenic inflammation and pain produced by bacterial endotoxins Gram-negative bacterial infections are accompanied by inflammation and somatic or visceral pain. These symptoms are generally attributed to sensitization of nociceptors by inflammatory mediators released by immune cells. Nociceptor sensitization during inflammation occurs through activation of the Toll-like receptor 4 (TLR4) signalling pathway by lipopolysaccharide (LPS), a toxic by-product of bacterial lysis. Here we show that LPS exerts fast, membrane delimited, excitatory actions via TRPA1, a transient receptor potential cation channel that is critical for transducing environmental irritant stimuli into nociceptor activity. Moreover, we find that pain and acute vascular reactions, including neurogenic inflammation (CGRP release) caused by LPS are primarily dependent on TRPA1 channel activation in nociceptive sensory neurons, and develop independently of TLR4 activation. The identification of TRPA1 as a molecular determinant of direct LPS effects on nociceptors offers new insights into the pathogenesis of pain and neurovascular responses during bacterial infections and opens novel avenues for their treatment. Gram-negative bacteria are a major class of human pathogens comprising many different virulent species [1] . Infections by these bacteria cause diseases that represent serious global health problems such as pneumonia, meningitis, gastroenteritis and gonorrhoea. The mammalian innate immune system uses a limited set of pattern-recognition receptors to trigger defence mechanisms against microbial infections [2] , [3] . The most potent immunostimulatory cue produced by Gram-negative bacteria is lipopolysaccharide (LPS), an abundant outer wall glycolipid that is released locally and into the circulation on bacterial lysis. In vertebrates, the lipid portion of LPS, termed lipid A, binds to the protein complex formed by MD-2 and Toll-like receptor 4 (TLR4) in immune cells. This triggers the synthesis of proinflammatory cytokines (tumour necrosis factor (TNF)-α, interleukin (IL)-1, IL-6) that, through the recruitment of macrophages and eosinophils, induce inflammation and pain, followed by eventual bacterial lysis and clearance [4] , [5] . However, the response of the immune system is relatively slow and cannot account for some of the immediate effects of LPS. For instance, tail-flick hyperalgesia starts a few minutes after intraperitoneal (i.p.) LPS injection [6] . Also, LPS produces a strong fall in blood pressure within minutes of injection, long before TNF-α is detectable in the circulation [7] . Interestingly, nociceptive and vascular responses to injected LPS are abrogated by section of visceral sensory afferents [6] , [8] , [9] implying a neural component that would act as a fast pathway in the LPS signalling mechanism. LPS can activate sensory neurons in culture [10] , [11] . Moreover, the recent identification of TLR4 in sensory neurons suggested that some of the rapid LPS effects could be mediated by direct stimulation of sensory afferents [10] , [11] , [12] . Nonetheless, no molecular mechanism has yet been put forward to relate TLR4 stimulation to the fast activation of sensory neurons. Here we use a combination of techniques, including electrical recordings of primary sensory neurons, the application of blockers of TLR4 signalling and behavioural testing in different transgenic mice, and obtained conclusive evidence that TRPA1-expressing peripheral sensory afferents are directly activated by LPS in a TLR4-independent manner. We also dissect out the molecular mechanisms linking LPS exposure to the activation of peptidergic sensory terminals and the development of acute neurogenic inflammation and pain. Collectively, these findings could lead to new strategies for the treatment of pain, inflammation and vascular shock during bacterial infections. LPS activates TRPA1-expressing nociceptors Using intracellular calcium imaging, we found that LPS extracted from Escherichia coli (10 μg ml −1 ) stimulated 17.8% (32/180) of wild-type (WT) mouse nodose (that is, vagal) sensory neurons innervating the viscera ( Fig. 1a,d ). Notably, nodose neurons isolated from Tlr4 knockout (KO) mice responded to LPS with similar incidence (32/136, P =0.26, Fisher’s exact test; Fig. 1b,d ) and amplitude ( P =0.6, unpaired t -test; Supplementary Fig. 1b ), thus excluding mediation of this effect by TLR4. Interestingly, the vast majority of WT and Tlr4 KO neurons that responded to LPS also responded to 100 μM cinnamaldehyde (CA) and 100 nM capsaicin ( Fig. 1a,b,e ), indicating that they are polymodal nociceptor neurons [13] , [14] , and raising the possibility that the neuronal response to LPS was mediated by the wide-spectrum chemo-nociceptor channel TRPA1 (refs 13 , 15 , 16 ). Indeed, we found that nodose neurons from Trpa1 KO mice responded to LPS with significantly lower incidence (6.6%, 14/212, P <0.001, Fisher’s exact test; Fig. 1c,d ) and amplitude than neurons obtained from WT animals ( P <0.01, unpaired t -test; Supplementary Fig. 1b ). Experiments using trigeminal (TG) sensory neurons yielded similar results, namely, a large overlap of the neuron populations sensitive to LPS and CA in the WT (89.3%, 50/56) and drastic reduction in the incidence (5/250, P <0.0001, Fisher’s exact test; Fig. 1d ) and amplitude ( P <10 −4 , unpaired t -test; Supplementary Fig. 1 ) of responses to LPS in Trpa1 KO mouse neurons compared with WT (56/394). Moreover, pre-application of the TRPA1 inhibitor HC-030031 (ref. 17 ) nearly abolished TG neuron responses to LPS (2/132, P <10 −4 , Fisher’s exact test; Fig. 1d ), while removal of the inhibitor unleashed LPS-induced responses (17/132) mainly in CA-sensitive neurons (16/17; Fig. 1d ). Notably, responses to LPS in nodose neurons of Trpv1 KO mice [18] were robust ( Supplementary Fig. 1a ) and nearly as frequent (25/187, P =0.25, Fisher’s exact test) as in WT mice ( Fig. 1d ), indicating that TRPV1 channels are not a primary target for LPS action in nociceptors. Responsiveness to LPS was dose-dependent and could be detected for concentrations as low as 100 ng ml −1 and 1 μg ml −1 for nodose ( Fig. 1e ) and TG neurons ( Fig. 1f ), respectively. At the highest concentration of LPS tested, the overlap between LPS and CA sensitivity was 67% for nodose and 78% for TG neurons. Also, it is noteworthy that, for concentrations up to 10 μg ml −1 LPS, responsive neurons belonged nearly exclusively to the TRPA1-positive population, while at higher concentrations the response to LPS extended to other populations. 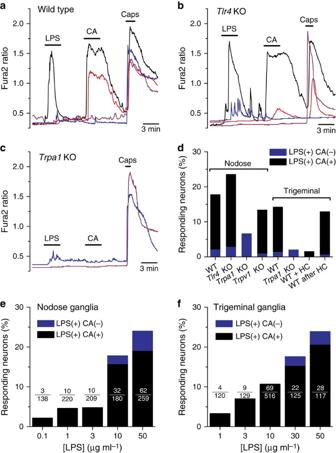Figure 1: TRPA1 mediates stimulation of nociceptor neurons by LPS. (a–c) Representative examples of the effects of LPS (10 μg ml−1) on [Ca2+]ilevels in nodose ganglion neurons isolated from WT (a),Tlr4KO (b) andTrpa1KO mice (c). Cinnamaldehyde (CA, 100 μM) and capsaicin (Caps, 100 nM) were applied to identify TRPA1- and TRPV1-expressing neurons, respectively. (d) Percentage of mouse nodose and TG sensory neurons responsive to LPS (blue) or to LPS and CA (black). The labels ‘WT+HC’ and ‘WT after HC’ refer to the responses to LPS (10 μg ml−1) observed in the presence of the TRPA1 inhibitor HC-030031 and after its removal, respectively. (e,f) Percentage of nodose (e) or TG (f) neurons responding to LPS (blue) or to LPS and CA (black) as a function of LPS concentration. Figure 1: TRPA1 mediates stimulation of nociceptor neurons by LPS. ( a – c ) Representative examples of the effects of LPS (10 μg ml −1 ) on [Ca 2+ ] i levels in nodose ganglion neurons isolated from WT ( a ), Tlr4 KO ( b ) and Trpa1 KO mice ( c ). Cinnamaldehyde (CA, 100 μM) and capsaicin (Caps, 100 nM) were applied to identify TRPA1- and TRPV1-expressing neurons, respectively. ( d ) Percentage of mouse nodose and TG sensory neurons responsive to LPS (blue) or to LPS and CA (black). The labels ‘WT+HC’ and ‘WT after HC’ refer to the responses to LPS (10 μg ml −1 ) observed in the presence of the TRPA1 inhibitor HC-030031 and after its removal, respectively. ( e , f ) Percentage of nodose ( e ) or TG ( f ) neurons responding to LPS (blue) or to LPS and CA (black) as a function of LPS concentration. Full size image LPS depolarizes TRPA1-expressing nociceptors Simultaneous monitoring of intracellular calcium levels and electrical activity in cell-attached mode revealed that calcium elevations caused by LPS in nodose neurons occurred during brief periods of action potential firing ( Fig. 2a ). Notably, excitatory effects of LPS on electrical activity were similar in WT and Tlr4 KO mice ( Fig. 2b ). During current-clamp recordings, a fraction (5/8) of cultured nodose neurons expressing TRPA1 channels depolarized rapidly (mean±s.e.m=16±4 mV), firing trains of action potentials in response to LPS ( Fig. 2c ). In contrast, these responses were not observed (0/10) ( P =0.006, Fisher’s exact test) in neurons insensitive to TRPA1 agonists ( Fig. 2c,d ). 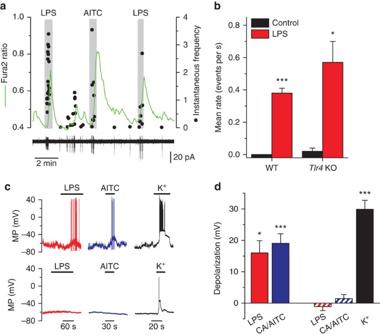Figure 2:E. coliLPS excites TRPA1-expressing sensory neurons. (a) Simultaneous recording of [Ca2+]ilevel (green trace) and instantaneous firing frequency (black dots) in cell-attached mode in a nodose neuron from aTlr4KO mouse. The large calcium transients (upper graph) during LPS and MO application correlate with the firing of action potentials (lower graph). (b) Summary results of effects ofE. coliLPS (10 μg ml−1) on mean±s.e.m. firing rate in nodose neurons from WT (n=4) andTlr4KO mice (n=3), (pairedt-test). WT neurons were electrically silent before LPS application. (c) Examples of recordings of membrane potential in the perforated-patch current-clamp mode (Ihold=0 pA) in two nodose neurons. LPS (10 μg ml−1) induces rapid depolarization and firing of action potentials in the TRPA1-expressing neuron (that is, AITC positive; upper traces). In contrast, LPS had no effect on membrane potential in the TRPA1-negative neuron (lower traces). (d) Average±s.e.m. depolarization of the resting membrane potential produced by LPS (n=5) and AITC (AITC) or CA (n=10) in TRPA1-expressing neurons (solid bars). The dashed bars represent the average depolarization produced by the application of LPS, AITC/CA or high extracellular potassium (60 mM) in neurons not expressing TRPA1 (n=10). Statistically significant differences of membrane potential (relative to control) are denoted by *P<0.05 and ***P<0.001, pairedt-test). Figure 2: E. coli LPS excites TRPA1-expressing sensory neurons. ( a ) Simultaneous recording of [Ca 2+ ] i level (green trace) and instantaneous firing frequency (black dots) in cell-attached mode in a nodose neuron from a Tlr4 KO mouse. The large calcium transients (upper graph) during LPS and MO application correlate with the firing of action potentials (lower graph). ( b ) Summary results of effects of E. coli LPS (10 μg ml −1 ) on mean±s.e.m. firing rate in nodose neurons from WT ( n =4) and Tlr4 KO mice ( n =3), (paired t -test). WT neurons were electrically silent before LPS application. ( c ) Examples of recordings of membrane potential in the perforated-patch current-clamp mode ( I hold =0 pA) in two nodose neurons. LPS (10 μg ml −1 ) induces rapid depolarization and firing of action potentials in the TRPA1-expressing neuron (that is, AITC positive; upper traces). In contrast, LPS had no effect on membrane potential in the TRPA1-negative neuron (lower traces). ( d ) Average±s.e.m. depolarization of the resting membrane potential produced by LPS ( n =5) and AITC (AITC) or CA ( n =10) in TRPA1-expressing neurons (solid bars). The dashed bars represent the average depolarization produced by the application of LPS, AITC/CA or high extracellular potassium (60 mM) in neurons not expressing TRPA1 ( n =10). Statistically significant differences of membrane potential (relative to control) are denoted by * P <0.05 and *** P <0.001, paired t -test). Full size image To analyse whether LPS acts on the peripheral terminals of primary sensory neurons expressing TRPA1, we recorded the impulse activity of TG nerve afferents innervating the mouse tongue ex vivo . Application of LPS onto the receptive field of sensory units, identified as nociceptive by their response to heat or capsaicin, produced a significant increase in the firing frequency in 50% of them, precisely those that were also activated by the TRPA1 agonist allyl isothiocyanate (AITC; Supplementary Fig. 2 ). This indicates that LPS activates the fraction of peripheral nociceptor fibres expressing TRPA1. Taken together, these results demonstrate that the chemosensitive cation channel TRPA1, but not the canonical LPS receptor TLR4, is critical for the acute excitatory effects of LPS on nociceptor sensory neurons. LPS activates TRPA1 channels Next, we determined whether LPS stimulates TRPA1 channels by measuring [Ca 2+ ] i changes in Chinese hamster ovary (CHO) cells expressing recombinant mouse TRPA1 channels (mTRPA1 cells) [13] . LPS induced a dose-dependent and reversible increase of [Ca 2+ ] i with an effective concentration of 3.3±0.5 μg ml −1 (mean±s.e.m for all values) ( Fig. 3a,b ). LPS did not induce Ca 2+ responses in Ca 2+ -free (plus 1 mM EGTA) solutions (ratio change=−0.0042±0.0008, n =46, P =1.0; paired t -test), or in non-transfected CHO cells ( Fig. 3a ), indicating that LPS induces Ca 2+ influx through mTRPA1 channels in the plasma membrane. Importantly, LPS also stimulated human embryonic kidney (HEK)-293 cells transfected with human TRPA1 ( Supplementary Fig. 3a ), but was ineffective, at 3 μg ml −1 , on three other human TRP channels known to be expressed in primary sensory neurons, namely, the vanilloid receptor TRPV1, the menthol receptor TRPM8 and the Δ9-tetrahydrocannabinol-activated receptor TRPV2 ( Supplementary Fig. 3b–d ). 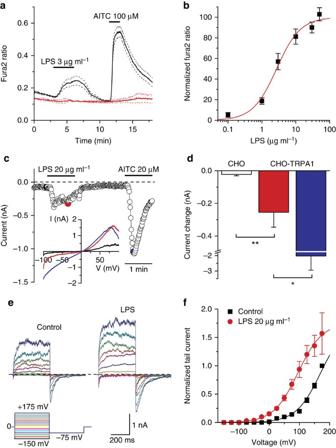Figure 3: LPS stimulates recombinant mouse TRPA1 channels. (a) Ratiometric [Ca2+]imeasurement showing the effect of LPS on mTRPA1 cells. Non-transfected cells (red traces) did not respond to LPS. The thick traces represent the means and the dashed traces represent the means±the corresponding s.e.m. (n≥25 cells for each trace). (b) Dose dependency of LPS-evoked [Ca2+]iresponses (mean±s.e.m.) (>80 cells per data point). The solid line represents the fit with a Hill equation. (c) Time course of TRPA1 current response to LPS (20 μg ml−1) and AITC (20 μM) monitored at −75 mV. The coloured data points correspond to the current traces shown in the inset. (d) Average±s.e.m. maximal amplitude of the currents (Tof recording=25 °C) during extracellular application of LPS (red bar) or AITC (blue bar) in mTRPA1 cells (n=7) and in control (white bar; CHO cells (n=6). Amplitude differences have been compared by an unpairedt-test. *P<0.05, **P<0.01. (e) Whole-cell currents in response to a double-pulse voltage protocol in control and in the presence ofE. coliLPS (20 μg ml−1), showing the increase in current amplitude and the slowing of channel closure. (f) Average±s.e.m. voltage dependence of TRPA1 peak tail current at −75 mV in control and in the presence of 20 μg ml−1LPS (n=6). Data were normalized to the value obtained at +175 mV in control. The solid lines represent the fit of the data with Boltzmann functions. Figure 3: LPS stimulates recombinant mouse TRPA1 channels. ( a ) Ratiometric [Ca 2+ ] i measurement showing the effect of LPS on mTRPA1 cells. Non-transfected cells (red traces) did not respond to LPS. The thick traces represent the means and the dashed traces represent the means±the corresponding s.e.m. ( n ≥25 cells for each trace). ( b ) Dose dependency of LPS-evoked [Ca 2+ ] i responses (mean±s.e.m.) (>80 cells per data point). The solid line represents the fit with a Hill equation. ( c ) Time course of TRPA1 current response to LPS (20 μg ml −1 ) and AITC (20 μM) monitored at −75 mV. The coloured data points correspond to the current traces shown in the inset. ( d ) Average±s.e.m. maximal amplitude of the currents ( T of recording=25 °C) during extracellular application of LPS (red bar) or AITC (blue bar) in mTRPA1 cells ( n =7) and in control (white bar; CHO cells ( n =6). Amplitude differences have been compared by an unpaired t -test. * P <0.05, ** P <0.01. ( e ) Whole-cell currents in response to a double-pulse voltage protocol in control and in the presence of E. coli LPS (20 μg ml −1 ), showing the increase in current amplitude and the slowing of channel closure. ( f ) Average±s.e.m. voltage dependence of TRPA1 peak tail current at −75 mV in control and in the presence of 20 μg ml −1 LPS ( n =6). Data were normalized to the value obtained at +175 mV in control. The solid lines represent the fit of the data with Boltzmann functions. Full size image Stimulation of mouse TRPA1 by LPS was confirmed in whole-cell patch-clamp recordings in mTRPA1 cells; extracellular application of LPS (20 μg ml −1 ) induced a significant increase in the amplitude of non-selective cation currents (reversal potential=−2.7±1.9 mV, n =7; Fig. 3c,d ). In contrast, LPS was ineffective in non-transfected CHO cells ( Fig. 3d , Supplementary Fig. 4a,b ). The maximal current increase induced by the potent TRPA1 agonist AITC (20 μM) was approximately eightfold larger than that elicited by 20 μg ml −1 LPS ( Fig. 3d ), indicating that LPS has lower efficacy. Moreover, pre-application of the TRPA1 inhibitor HC-030031 fully prevented the activating effects of LPS ( n =5). The inhibition of TRPA1 whole-cell current by HC-030031 was reversible on wash and could be reinstated on reapplication of the blocker ( Supplementary Fig. 4c ). At −75 mV, current density averaged −8.2±1.7 pA pF −1 in HC-030031 plus LPS and −39.4±6.5 pA pF −1 after HC-030031 wash ( n =7, P <0.001, paired t -test). Next, we explored the mechanism(s) through which LPS stimulates TRPA1. LPS could potentially activate TRPA1 by modulating [Ca 2+ ] i (refs 19 , 20 ). However, LPS was able to stimulate TRPA1 in Ca 2+ -free conditions ( Fig. 3e , Fig. 4 ). Alternatively, TRPA1 could be activated by an endogenous electrophilic compound that could be eventually produced on LPS application. However, LPS induced a significant activation of the AITC-insensitive TRPA1-mutant C622S in HEK-293 cells (increase in Fura-2 ratio of 0.38±0.03, n =36, P <0.01, paired t -test). Analysis of the macroscopic TRPA1 currents activated by LPS in Ca 2+ -free conditions indicated a slowing of channel deactivation, an acceleration of channel opening ( Fig. 3e , Supplementary Fig. 5 ) and a concomitant leftward shift in the voltage dependence of channel activation ( Fig. 3f ). These data demonstrate that, as occurs with other TRPA1 activators [21] , [22] , LPS acts as a gating modifier of TRPA1, destabilizing the closed state(s) and stabilizing the open conformation(s). 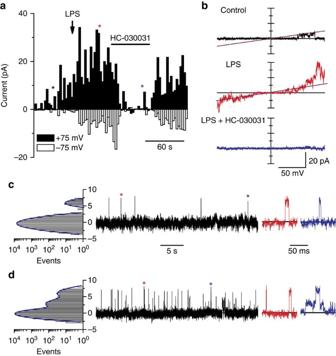Figure 4: LPS activates TRPA1 channels in a membrane-delimited manner. (a) Time course of current amplitudes recorded in outside-out patches of TRPA1-expressing CHO cells at –75 and +75 mV. Currents were elicited by voltage ramps from −100 to +100 mV from a holding potential of 0 mV. The arrow indicates the moment of application of LPS (10 μg ml−1) and the horizontal bar indicates the period of exposure to 50 μM HC-030031. The coloured asterisks mark the time points at which the corresponding current traces shown inbwere recorded. Single-channel records in the outside-out configuration at +75 mV, in control solution (c) and in the presence of 10 μg ml−1LPS (d). Events marked with an asterisk are displayed at an expanded timescale. The histograms on the left show the corresponding distributions of the current amplitudes. All records in the figure were obtained in Ca2+-free conditions. Figure 4: LPS activates TRPA1 channels in a membrane-delimited manner. ( a ) Time course of current amplitudes recorded in outside-out patches of TRPA1-expressing CHO cells at –75 and +75 mV. Currents were elicited by voltage ramps from −100 to +100 mV from a holding potential of 0 mV. The arrow indicates the moment of application of LPS (10 μg ml −1 ) and the horizontal bar indicates the period of exposure to 50 μM HC-030031. The coloured asterisks mark the time points at which the corresponding current traces shown in b were recorded. Single-channel records in the outside-out configuration at +75 mV, in control solution ( c ) and in the presence of 10 μg ml −1 LPS ( d ). Events marked with an asterisk are displayed at an expanded timescale. The histograms on the left show the corresponding distributions of the current amplitudes. All records in the figure were obtained in Ca 2+ -free conditions. Full size image LPS activates TRPA1 channels in a membrane-delimited manner To gain further insight into the mechanism of TRPA1 activation by LPS, we performed patch-clamp recordings in cell-free outside-out patches in the absence of intracellular and extracellular Ca 2+ . Under these conditions, extracellular application of LPS enhanced TRPA1 currents (6.1±1.6-fold increase at −75 mV; P =0.018, n =5, paired t -test; Fig. 4a,b ). The single-channel conductance, estimated from linear fits to currents evoked during voltage ramps, was nearly identical in control and in the presence of LPS (96±3 pS and 94±2 pS, respectively; n =5, Fig. 4b ), and the TRPA1 antagonist HC-030031 induced a powerful inhibition of LPS-induced single-channel currents (97±2%, n =5, Fig. 4a,b ). In outside-out patches held at +75 mV, with Ca 2+ -free extracellular and intracellular solutions, the basal open probability was on average 0.014±0.004 ( Fig. 4c ), while mean closed time and mean open time were 2.0±1.2 s and 8.1±1.0 ms, respectively, ( n =5). In these patches, LPS induced a 5.7±1.6-fold increase in the open probability ( P =0.023), a 4±1-fold reduction of the mean closed time ( P =0.0016) and a 1.8±0.4-fold increase in the mean open time ( P =0.04; n =5, paired t -test; Fig. 4d ). Of note, we recorded half-sized openings, which may reflect the incidence of subconductance open state(s). LPS and endogenous TRPA1 agonists have synergistic effects One fundamental aspect of TRPA1 function is to act as molecular integrator for multiple irritants and inflammatory mediators [15] , [23] . Thus, it was important to determine whether the effects of LPS on TRPA1 could be potentiated by other algesic compounds. At sites of infection and inflammation, various endogenous molecules are generated that could sensitize the response of TRPA1 to LPS. In particular, inflammation increases the local levels of 4-hydroxy-2-nonenal (HNE) and other lipid peroxidation products that are potent stimulators of TRPA1 (refs 24 , 25 ). Thus, we hypothesized that LPS and HNE may act synergistically on TRPA1. Indeed, the co-application of low concentrations of HNE and LPS produced a strong potentiation of TRPA1 activity, resulting in much larger currents than the sum of each agonist applied alone ( Supplementary Fig. 6 ). As expected for a TRPA1-dependent effect, these currents were fully suppressed by HC-030031 ( Supplementary Fig. 6 ). The shape of lipid A determines TRPA1 activation by LPS Suspecting that LPS insertion in the plasma membrane is responsible for its stimulatory action on TRPA1 channels, we tested the effect of lipid A, the membrane-anchored lipid moiety of LPS [26] . Application of 50 μg ml −1 diphosphoryl lipid A from E. coli induced [Ca 2+ ] i responses in mTRPA1 cells, but not in control cells ( Fig. 5a ). Moreover, application of lipid A to nodose neurons produced robust Ca 2+ elevations exclusively in a subpopulation (9/41, 22%) of CA-activated neurons ( Fig. 5b ). Interestingly, synthetic monophosphoryl lipid A also activated mTRPA1 cells ( Supplementary Fig. 7 ) ruling out a biological contaminant during LPS purification as a possible source of the effect. 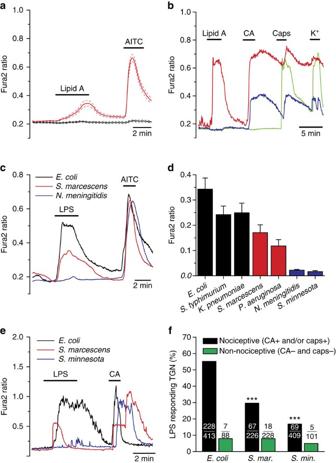Figure 5: The shape of lipid A determines TRPA1 activation by LPS. (a) Ratiometric [Ca2+]iimaging experiment showing the effect of extracellular application of lipid A on CHO mTRPA1 cells. Thirty-six percent of the TRPA1-expressing cells (AITC-sensitive) responded to lipid A (red traces,n=50). Non-transfected cells (black traces) did not respond to lipid A (n=20). Solid and broken traces represent mean and ±s.e.m., respectively. (b) Representative responses of mouse nodose neurons to lipid A, CA (100 μM), capsaicin (1 μM) and high K+(30 mM). A fraction of CA-sensitive neurons was also activated by lipid A. (c) Mean [Ca2+]ielevation evoked by LPS extracted fromE. coli,S. marcescensandN. meningitidis(20 μg ml−1) in mTRPA1 cells (n>25 for each trace). (d) Average±s.e.m. amplitude of [Ca2+]ievoked by LPSs with different lipid A conformation in mTRPA1 cells (n=26–129). (e) Representative examples of responses in TG neurons to different types of LPS. (f) Percentage of TG neurons responding to different types of LPS. In nociceptive neurons, responses toS. marcescensandS. minnesotaLPS were significantly reduced (***P<0.001) compared withE. coli(Fisher’s exact test). In non-nociceptive neurons, responses were not different. Figure 5: The shape of lipid A determines TRPA1 activation by LPS. ( a ) Ratiometric [Ca 2+ ] i imaging experiment showing the effect of extracellular application of lipid A on CHO mTRPA1 cells. Thirty-six percent of the TRPA1-expressing cells (AITC-sensitive) responded to lipid A (red traces, n =50). Non-transfected cells (black traces) did not respond to lipid A ( n =20). Solid and broken traces represent mean and ±s.e.m., respectively. ( b ) Representative responses of mouse nodose neurons to lipid A, CA (100 μM), capsaicin (1 μM) and high K + (30 mM). A fraction of CA-sensitive neurons was also activated by lipid A. ( c ) Mean [Ca 2+ ] i elevation evoked by LPS extracted from E. coli , S. marcescens and N. meningitidis (20 μg ml −1 ) in mTRPA1 cells ( n >25 for each trace). ( d ) Average±s.e.m. amplitude of [Ca 2+ ] i evoked by LPSs with different lipid A conformation in mTRPA1 cells ( n =26–129). ( e ) Representative examples of responses in TG neurons to different types of LPS. ( f ) Percentage of TG neurons responding to different types of LPS. In nociceptive neurons, responses to S. marcescens and S. minnesota LPS were significantly reduced (*** P <0.001) compared with E. coli (Fisher’s exact test). In non-nociceptive neurons, responses were not different. Full size image The intrinsic conformation of lipid A is critical for LPS bioactivity (for example, induction of cytokine production), with conical shapes conferring more activity than cylindrical ones [27] , [28] . This conformation is largely determined by the number of charged phosphate groups and acyl chains, and varies among different bacterial strains [26] . We found that LPSs with asymmetrical hexa-acyl lipid A ( E. coli, Salmonella typhimurium and Klebsiella pneumoniae ) induced the strongest TRPA1 responses ( Fig. 5c,d ). In comparison, LPSs with asymmetrical penta-acyl lipid A ( Serratia marcescens , Pseudomonas aeruginosa ) induced smaller effects on TRPA1. Finally, LPS from Neisseria meningitidis , with symmetrical hexa-acyl lipid A, and from S. minnesota , which is known to form symmetrical lamellar structures, had virtually no effect on TRPA1. Very similar results were obtained in cultured TG neurons: the percentage of neurons responding to LPS followed the sequence ( E. coli > S. marcescens > S. minnesota ) and the great majority of LPS responders had a nociceptive phenotype ( Fig. 5e,f ). These results strongly suggest that the capacity of a given LPS to activate TRPA1 correlates with its ability to induce mechanical alterations in the plasma membrane. We also found that trinitrophenol (TNP), a negatively charged amphiphatic compound inducing mechanical tension of the lipid membrane, and known to modulate the gating of mechanosensitive channels [29] , including TRPA1 (ref. 30 ) also potentiated LPS activity. Pretreatment with TNP strongly potentiated [Ca 2+ ] i responses to low concentrations of LPS in mTRPA1 cells ( Supplementary Fig. 8a–d ). LPS effects on TRPA1 are TLR4 independent Generally, LPS effects on neurons have been linked to activation of the TLR4 signalling pathway [10] . However, as shown earlier, we found that the excitatory effects of LPS were still observed on sensory neurons isolated from Tlr4 KO mice. We also tested CLI-095, a novel specific inhibitor of TLR4 signalling [31] . As shown in Fig. 6a–c , pretreatment for 10 min with 1 μM CLI-095 did not affect the subsequent response to LPS in nodose neurons; neither the percentage of responding neurons nor the amplitude of the response was significantly affected. Similar results were obtained in TRPA1-expressing CHO cells ( Supplementary Fig. 9 ). In addition, CHO cells transfected with human TLR4 did not show a TRPA1-like current when acutely exposed to LPS ( Supplementary Fig. 10 ). Altogether, these results strongly support a TLR4-independent mechanism of action of LPS on TRPA1 channels. 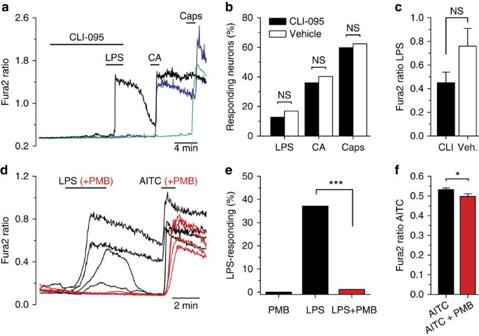Figure 6: The effects of LPS on TRPA1 channels are independent of TLR4 signalling and require lipid A activity. (a) Representative example of responses to LPS in nodose neurons following preincubation for 10 min with CLI-095 (1 μM). (b) The percentage of neurons responding to LPS, CA or capsaicin was not affected by preincubation with CLI-095 (n=189) compared with vehicle (n=77), Fisher’s exact test. (c) Mean±s.e.m. amplitude of the response to LPS in CLI-095 (n=24) and vehicle (n=13) was not significantly different (unpairedt-test). (d) Preincubation (30 min) of LPS (3 μg ml−1) with polymyxin B (PMB; 300 ng ml−1) abrogated responses in mTRPA1 cells to LPS. The same incubation had minimal effects on the response to AITC (100 μM). (e) Percentage of CHO-TRPA1 cells responding to PMB, LPS or LPS+PMB (n>50 cells). The inhibition of LPS responses was highly significant (Fischer’s exact test). (f) The amplitude of calcium response to MO was minimally reduced by PMB (mean±s.e.m.,n>100 cells). Figure 6: The effects of LPS on TRPA1 channels are independent of TLR4 signalling and require lipid A activity. ( a ) Representative example of responses to LPS in nodose neurons following preincubation for 10 min with CLI-095 (1 μM). ( b ) The percentage of neurons responding to LPS, CA or capsaicin was not affected by preincubation with CLI-095 ( n =189) compared with vehicle ( n =77), Fisher’s exact test. ( c ) Mean±s.e.m. amplitude of the response to LPS in CLI-095 ( n =24) and vehicle ( n =13) was not significantly different (unpaired t -test). ( d ) Preincubation (30 min) of LPS (3 μg ml −1 ) with polymyxin B (PMB; 300 ng ml −1 ) abrogated responses in mTRPA1 cells to LPS. The same incubation had minimal effects on the response to AITC (100 μM). ( e ) Percentage of CHO-TRPA1 cells responding to PMB, LPS or LPS+PMB ( n >50 cells). The inhibition of LPS responses was highly significant (Fischer’s exact test). ( f ) The amplitude of calcium response to MO was minimally reduced by PMB (mean±s.e.m., n >100 cells). Full size image We took additional steps to verify that activation of TRPA1 was truly mediated by LPS. To minimize the possible role of a contaminant, we tested ultrapure forms of LPS (see Methods ). As shown in Supplementary Fig. 11 , ultrapure LPS from E. coli (2 μg ml −1 ) also activated TRPA1-expressing cells. Moreover, the ultrapure form of S. minnesota R595, at a 10 times higher concentration, showed almost no response, similar to the results obtained from a different source (see Fig. 5c,d ). Strikingly, an ultrapure LPS from Rhodobacter sphaeroides , which acts as a competitive antagonist of TLR4 (ref. 32 ), also activated TRPA1-expressing cells ( Supplementary Fig. 11 ), strongly suggesting a TLR4-independent mechanisms of action. In contrast, the same preparations of LPS had the expected effects on human TLR4 signalling ( Supplementary Fig. 11d ). Polymyxin B is a cationic cyclic polypeptide antibiotic that is widely used to neutralize the effects of endotoxin contamination in biological samples [33] . The action of polymyxin B is based on its binding, by electrostatic interaction, to the anionic lipid A. Incubation of LPS with polymyxin B completely eliminated the activation of TRPA1 by LPS ( Fig. 6d,e ). In contrast, activation of TRPA1 by AITC was minimally reduced ( Fig. 6f ). This result suggests that the inhibitory action of polymyxin B is not directly on the channel (for example, pore block) and further implicates lipid A in the effects observed. Acute neuropeptide release by LPS depends on TRPA1 activity TRPA1 participates in neurogenic inflammation and vasodilation [34] , [35] , [36] . To test whether activation of peptidergic sensory terminals by LPS leads to neuropeptide release and neurogenic inflammation [14] , [37] , we used an isolated mouse trachea preparation. The trachea is densely innervated with peptidergic vagal fibres that release calcitonin gene-related peptide (CGRP) in response to capsaicin [38] , [39] . Brief incubation of tracheal halves with acrolein, an electrophilic TRPA1 activator and product of oxidative stress, also present in fumes and as a toxic metabolite of chemotherapy agents [15] , produced a dose-dependent release of CGRP ( Supplementary Fig. 12 ). Application of LPS (30–100 μg ml −1 ) to tracheal halves induced a modest but significant CGRP release ( Fig. 7a ). In addition, a brief pretreatment of the trachea with the membrane crenator TNP produced a massive potentiation of the CGRP release evoked by LPS ( P <10 −4 ) and by acrolein ( P <0.01; Fig. 7a ). Notably, responses to individual agonists, or potentiated response to LPS in the presence of TNP were fully abrogated in Trpa1 KO mouse tracheas ( Fig. 7a ), indicating that they depend strictly on activation of TRPA1 channels. We also observed a fourfold potentiation of CGRP release from the trachea by LPS in the presence of the endogenous TRPA1 agonist HNE ( Fig. 7b ), fully consistent with the synergistic action of both agonists on TRPA1 whole-cell currents as we have shown ( Supplementary Fig. 6 ). Collectively, these results indicate that LPS, both alone and in combination with other endogenous inflammatory mediators, can activate TRPA1 in sensory nerve terminals leading to acute neurogenic inflammation. 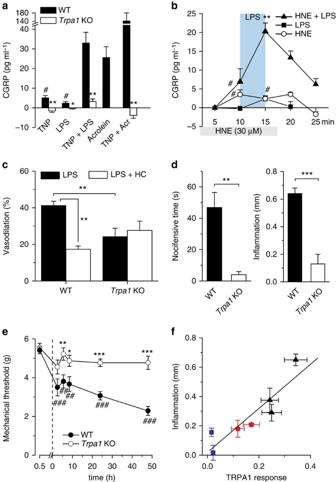Figure 7: Neurogenic inflammation and pain by LPS depend on TRPA1 activity. (a) Trinitrophenol (TNP, 50 μM) and LPS (100 μg ml−1) evoke (mean±s.e.m.) modest but significant (#P<0.05, Wilcoxon test,n=12/8) tracheal CGRP release; preincubation with TNP potentiates response to LPS and acrolein (30 μM).Trpa1KO mice do not respond to LPS (*P<0.05, analysis of variance (ANOVA) Fisher’s least significant difference (LSD) test,n=4), TNP or its co-application with LPS or acrolein (**P<0.01). (ANOVA Fisher’s LSD test,n=8, 4, 4). (b) LPS and 4-hydroxy-2-nonenal (HNE) evoke small but significant (#P<0.05) CGRP responses. Preincubation with low concentration of HNE potentiates tracheal CGRP release evoked by LPS (**P<0.01, ANOVA Fisher’s LSD test,n=4, mean±s.e.m.). (c) Summary of effect of LPS (100 μg ml−1) perfusion on mesenteric artery diameter (mean±s.e.m.) from WT (n=7) andTrpa1KO (n=8) mice in control condition and in the presence of HC-030031 (10 μM). Arteries precontracted with the alpha1 adrenergic agonist phenylephrine (2 μM). Statistical differences were evaluated with an unpairedt-test. (d) The nocifensive response and the acute local inflammation produced by intraplantar LPS injection (5 μg μl−1in 10 μl) were nearly abolished inTrpa1KO animals (n=6) compared with WT littermates (n=7) (unpairedt-test, values are mean±s.e.m.). (e) Mechanical paw withdrawal threshold (mean±s.e.m.) to mechanical stimulation before and after intraplantar injection of LPS (5 μg μl−1) in WT (n=14) andTrpa1KO (n=14) animals. The asterisks reflect the differences in threshold between WT and KO (unpairedt-test). Comparison between baseline and the different time points gave significant differences (##P<0.01,###P<0.001) in WT animals only (one-way ANOVA with Bonferroni’s correction). (f) Correlation between the hind paw inflammation (mean±s.e.m.) induced by LPSs of different shapes (blue for cylindrical, red for semiconical and black for conical;n=5–9) with the potency for TRPA1 activation (mean±s.e.m.) estimated from the amplitude of Ca2+response evoked in mTRPA1 cells;Fig. 5d). Figure 7: Neurogenic inflammation and pain by LPS depend on TRPA1 activity. ( a ) Trinitrophenol (TNP, 50 μM) and LPS (100 μg ml −1 ) evoke (mean±s.e.m.) modest but significant ( # P <0.05, Wilcoxon test, n =12/8) tracheal CGRP release; preincubation with TNP potentiates response to LPS and acrolein (30 μM). Trpa1 KO mice do not respond to LPS (* P <0.05, analysis of variance (ANOVA) Fisher’s least significant difference (LSD) test, n =4), TNP or its co-application with LPS or acrolein (** P <0.01). (ANOVA Fisher’s LSD test, n =8, 4, 4). ( b ) LPS and 4-hydroxy-2-nonenal (HNE) evoke small but significant ( # P <0.05) CGRP responses. Preincubation with low concentration of HNE potentiates tracheal CGRP release evoked by LPS (** P <0.01, ANOVA Fisher’s LSD test, n =4, mean±s.e.m.). ( c ) Summary of effect of LPS (100 μg ml −1 ) perfusion on mesenteric artery diameter (mean±s.e.m.) from WT ( n =7) and Trpa1 KO ( n =8) mice in control condition and in the presence of HC-030031 (10 μM). Arteries precontracted with the alpha1 adrenergic agonist phenylephrine (2 μM). Statistical differences were evaluated with an unpaired t -test. ( d ) The nocifensive response and the acute local inflammation produced by intraplantar LPS injection (5 μg μl −1 in 10 μl) were nearly abolished in Trpa1 KO animals ( n =6) compared with WT littermates ( n =7) (unpaired t -test, values are mean±s.e.m.). ( e ) Mechanical paw withdrawal threshold (mean±s.e.m.) to mechanical stimulation before and after intraplantar injection of LPS (5 μg μl −1 ) in WT ( n =14) and Trpa1 KO ( n =14) animals. The asterisks reflect the differences in threshold between WT and KO (unpaired t -test). Comparison between baseline and the different time points gave significant differences ( ## P <0.01, ### P <0.001) in WT animals only (one-way ANOVA with Bonferroni’s correction). ( f ) Correlation between the hind paw inflammation (mean±s.e.m.) induced by LPSs of different shapes (blue for cylindrical, red for semiconical and black for conical; n =5–9) with the potency for TRPA1 activation (mean±s.e.m.) estimated from the amplitude of Ca 2+ response evoked in mTRPA1 cells; Fig. 5d ). Full size image Neurovascular responses to LPS involve activation of TRPA1 Systemic bacterial invasion can cause massive peripheral vasodilation, leading to a severe drop in blood pressure, a life-threatening condition known as septic shock [40] . Considering that chemical stimulation of TRPA1 in sensory fibres innervating resistance arteries induces potent vasodilation [24] , [34] , [35] , [36] , we tested whether this channel was involved in the vascular response to LPS. Using pressure myography ex vivo , we found that LPS (100 μg ml −1 ) induced a strong dilation in WT mouse mesenteric arteries precontracted with the alpha1 adrenergic agonist phenylephrine (2 μM; Fig. 7c and Supplementary Fig. 13a ). Notably, this effect was significantly reduced by the specific TRPA1 inhibitor HC-030031 (10 μM) and by genetic ablation of TRPA1 ( Fig. 7c and Supplementary Fig. 13b ). Moreover, in Trpa1 KO animals, the residual LPS-induced dilation was completely insensitive to HC-030031 ( Fig. 7c and Supplementary Fig. 13b ). Thus, TRPA1 appears to participate in the vasodilation response to LPS, although other yet unidentified targets also appear to contribute to the arterial vasomotor responses. Acute LPS-induced hypersensitivity engages TRPA1 but not TLR4 The typical symptoms of local Gram-negative bacterial infections include inflammation, pain and mechanical hypersensitivity [41] , [42] . They were readily reproduced experimentally with intraplantar injections of purified E. coli LPS in WT mice ( Fig. 7d,e ). Consistent with a major role of TRPA1 as a LPS effector, we found that such responses were severely attenuated in Trpa1 KO mice ( Fig. 7d,e ). A similar attenuation of mechanical hyperalgesia to LPS injection in Trpa1 KO mice was reported recently [43] . Moreover, the local inflammation caused by LPS molecules with different lipid A shape was strongly correlated with their ability to stimulate mTRPA1 in vitro ( r =0.91, P <0.01; Fig. 7f ) linear correlation coefficient ( n =7). In contrast, acute pain responses, local tissue swelling and mechanical hyperalgesia developed normally in Tlr4 KO mice following LPS injection ( Supplementary Fig. 14 ). Notably, mechanical hyperalgesia resolved more rapidly in Tlr4 KO mice compared with wild type, suggesting that immune response pathways are engaged by LPS in a slower timescale compared with TRPA1 activation. TRPA1 is not critical for LPS systemic inflammatory response As deletion of TRPA1 produces such prominent effects on nociceptive and neurovascular response to LPS, we wondered whether other, well-established, systemic responses to LPS were affected as well. In mice, i.p. application of high doses of LPS produces a profound and long-lasting hypothermia [44] . As previously described, the injection of 3 mg kg −1 E. coli LPS produced a marked hypothermia in WT mice ( Supplementary Fig. 15 ). The severity and time course of this hypothermic response was nearly identical in Trpa1 KO littermates. Activation of TLR4 by LPS is known to potently activate immune cells (for example, hepatic macrophages) to produce and release proinflammatory cytokines such as TNF-α and IL-6 (refs 4 , 45 ). Indeed, i.p. LPS treatment (0.75 and 1 mg kg −1 for 1 h) increased dose dependently circulating serum IL-6 levels from an undetectable baseline after saline injection ( Supplementary Fig. 16a ). As was the case for thermoregulatory responses, we did not find differences in the levels of IL-6 between both genotypes of mice. Moreover, LPS treatment (1 mg kg −1 for 1 h) also increased IL-6 messenger RNA levels in the liver in both types of mice similarly ( Supplementary Fig. 16b ). Here we demonstrate that TRPA1 channels are key participants in the biological response to LPS, a microbial signature molecule, translating the presence of elevated LPS into a rapid nociceptor response and neurogenic inflammation. Therefore, LPS appears as a totally novel class of biological toxin among the large number of natural compounds that are detected by TRPA1 channels (reviewed by Nilius et al . [16] ). The ancient nature of LPS and the fact that the role of TRPA1 in chemical avoidance is conserved from flies to mammals underscores the evolutionary significance of this alert mechanism in animals [14] , [46] , [47] , [48] . It is noteworthy that bacterial sepsis is accompanied by severe redox imbalance, favouring the oxidant state [49] , a condition that also leads to robust TRPA1 channel activation [24] , [50] . Our findings also raise the question of how this channel can function as such an extremely broadly tuned chemo-nocisensor. In the light of previous studies and of the present results, it seems clear that rather than using specific molecular determinants (that is, the key and lock concept), TRPA1 activation relies on the general physico-chemical properties of the agonist. Whereas highly reactive electrophilic irritants are detected by their capacity to modify covalently key amino-acid residues in the amino terminus of the TRPA1 channel [47] , [51] , our results suggest that LPS modulates TRPA1 activity by inducing mechanical perturbations in the plasma membrane. This result is in line with the known mechanosensing function of TRPA1 in visceral [52] and somatic [53] , [54] neurons. The activation of TRPA1 by LPS in cell-free membrane patches indicates that the mechanism underlying this effect does not require other intermediate molecules, but additional experiments, including the characterization of LPS action after incorporation of TRPA1 into artificial lipid bilayers of defined composition, are needed to substantiate this point. Nevertheless, it is noteworthy that different forms of LPS activated TRPA1 in proportion to their ability to produce inflammation in vivo , which suggests a close relation between both processes. Recently, Hardie and Franze [55] showed, in a very elegant way, that activation of light-sensitive TRP and TRPL channels in Drosophila photoreceptors is mediated by rapid mechanical perturbation of the plasma membrane caused by phosphatidylinositol 4,5-bisphosphate (PIP 2 ) depletion downstream of PLC activation by light. This study is very relevant to the hypothetical activation of TRPA1 under pathophysiological conditions because TRPA1 is also activated by G-protein-coupled receptors that activate PLC and deplete PIP 2 (refs 15 , 23 ). In the context of infection, the production of some inflammatory mediators (for example, bradykinin and trypsin) that couple to Gq/11 will also lead to PIP 2 depletion. Thus, the mechanical perturbations produced by LPS hypothesized in our study could act synergistically with those produced by changes in PIP 2 levels, leading to TRPA1 gating. Sensory neurons express a number of TLR4 signalling elements, including TLR4, making it plausible that TLR4 signalling participates in sensory responses to LPS [11] . Indeed, several recent studies have implicated TLR4 in rapid responses to LPS in sensory neurons, including the sensitization of TRPV1 channels [10] . However, a number of results clearly indicate that TLR4 is dispensable for the excitatory actions of LPS on TRPA1. First and foremost, responses in sensory neurons from Tlr4 KO mice were indistinguishable from those observed in WT animals. Second, incubation with a specific inhibitor of TLR4 signalling did not affect responses to LPS in TRPA1-expressing neurons or recombinant TRPA1 channels. Moreover, acute pain and tissue swelling peaked normally in Tlr4 KO mice in vivo . Obviously, under in vivo conditions, circulating LPS will engage the available TLR4 machinery, including the production of proinflammatory cytokines, which could participate in the slow sensitization of nociceptors. Consistent with this view, we observed a faster resolution of the mechanical hypersensitivity, following local LPS injection, in Tlr4 KO mice. In vivo , we envision both effector pathways of LPS acting synergistically on somatic and visceral neurons. Our observation that LPS excites somatic and visceral nociceptor neurons via a mechanism dependent on TRPA1 activation and independent of TLR4 can readily explain acute pain and neurogenic inflammation induced by LPS. Similar concentrations of LPS have been used to evoke pain behaviour in experimental animals [42] . The activation of TLR4 occurs at lower LPS levels than those required to activate TRPA1 channels. However, severe endotoxemia can bring plasma LPS levels into the micromolar range [56] , levels also encountered in urine and locally inflamed tissues [57] . Moreover, we found strong (that is, 10-fold) potentiation of LPS-induced activation of TRPA1 by other TRPA1 agonists, including endogenous modulators (for example, HNE), suggesting that in the context of a bacterial infection in vivo , the levels of LPS required to activate TRPA1 may be lower than what we found experimentally. It should be noted that the ex vivo preparations we used (that is, the superfused trachea and the isolated tongue), in contrast to the skin in vivo , cannot reflect secondary inflammatory reactions, like plasma extravasation, accumulation of inflammatory mediators (for example, bradykinin, thrombocytes and immune cells), which, together, may complement or amplify, like we found with HNE or acrolein, the excitatory effects of LPS on TRPA1 to activate nociceptors [58] . The modest but significant effect of LPS alone on tracheal CGRP release is not surprising, because even prostaglandin E2, the most widely acknowledged nociceptor sensitizer, shows no effect of its own on nociceptor discharge and CGRP release but ‘only’ facilitates heat and chemical responses [59] . Finally, these avascular ex vivo preparations cannot be compared directly with dissociated sensory neurons in culture with respect to chemosensitivity, because the nerve endings do not reach the very surface of the mucosa, formed by epithelial cells and their tight junctions. TRPA1-mediated calcium influx in sensory terminals leads to release of neuropeptides [13] , [24] , thereby triggering rapid TRPA1-dependent vasodilation, local inflammation and sustained mechanical hyperalgesia. Recently, it was established that TRPA1-mediated substance P release in the colon plays a necessary role in experimental colitis [60] , providing further support for a causal link between TRPA1 channels and neuroimmune processes. Other studies have indicated the essential role of TRPA1 in the pathophysiology of asthma [37] , a disease with a significant immunological component. We found that in the absence of TRPA1 the proinflammatory and pro-algesic actions of LPS are severely curtailed. Interaction of LPS with the MD-2–TLR4 complex leading to activation of the transcription factor nuclear factor-kappaB (NF-κB) and cytokine production is the canonical pathway of LPS signalling [2] . The identification of TRPA1 as a functional target for LPS may represent an important missing link between the stimulation of afferent sensory fibres and the immune responses during a bacterial challenge. We tentatively conclude that TRPA1 channels and pattern receptors like TLR4 act as synergic sensory mechanisms, alerting the host about the presence of pathogens, allergens and environmental irritants [3] . TRPA1 would be involved in the early steps of the response cascade, sensing potentially damaging compounds, in parallel with the well-established production of proinflammatory cytokines. The recent discovery of activation of the NF-κB signalling pathway following TRPA1 activation provides independent support to our view [61] . Thus, identification of TRPA1 as a new target for LPS opens novel avenues for the treatment of adverse biological responses of Gram-negative bacterial infections. Finally, the recent report describing the activation of nociceptors by N -formylated peptides and the pore-forming toxin α−haemolysin isolated from bacteria, by mechanisms independent of immune pathways [62] , suggests that direct activation of nociceptors by bacterial products may be a more general signalling mechanism than previously recognized. Animals Experiments were performed in accordance with the guidelines established by the European Communities Council Directive (86/609/ECC), by Spanish Royal Decree 1201/2005 and the Ethics Committee of the Catholic University, Leuven. : Tlr4 KO mice on a C57BL/6 background, originally generated by Hoshino et al . [63] were kindly provided by C Guerri Centro de Investigación Príncipe Felipe (CIPF) and by H Hammad and B Lambrecht (VIB, Ghent, Belgium). Trpa1 KO mice were provided by D Corey [64] . Trpv1 KO mice, originally generated in D Julius laboratory [18] , were obtained from Jackson. Neuronal culture Neuronal culturing methods were similar to those used previously [65] , [66] . TG and nodose ganglia were isolated from young adult male mice (postnatal months 1–3), WT and Trpa1 KO siblings [64] , Tlr4 KO (ref. 63 ) and Trpv1 KO (ref. 18 ), and incubated for 1 h with 0.07% collagenase XI+0.3% Dispase at 37 °C. Thereafter, ganglia were mechanically dissociated and cultured in minimal essential medium with Earle’s balanced salt solution and L -Glutamine (Invitrogen) supplemented with 10% fetal bovine serum (Invitrogen), 1% minimal essential medium vitamin solution (Invitrogen), 100 μg ml −1 penicillin/streptomycin and 100 ng ml −1 nerve growth factor (NGF). Cells were plated on poly- L -lysine-coated glass coverslips and used after 1 day in culture. Cell culture CHO-K1 cells, from the American Type Culture Collection, were cultured in DMEM containing 10% of fetal bovine serum, 2% glutamax (Invitrogen), 1% non-essential amino acids (Invitrogen) and 200 μg ml −1 penicillin/streptomycin. An inducible CHO-K1 cell line stably expressing mouse TRPA1 channels was kindly provided by Ardem Patapoutian (The Scripps Research Institute, USA) [13] and cultured as detailed for the parental cell line. Expression of TRPA1 was induced by application of 0.25–0.5 μg ml −1 tetracycline 4–18 h before recording. HEK-293 cells, from the European Collection of Cell Cultures (Salisbury, UK), were seeded in 18 mm glass coverslips coated with poly- L -lysine (0.1 mg ml −1 ) and grown in DMEM containing 10% (v/v) human serum, 2 mM L -glutamine, 2 U ml −1 penicillin and 2 mg ml −1 streptomycin at 37 °C in a humidity-controlled incubator with 10% CO 2 . Human TRPA1, TRPV1, TRPM8 and TRPV2 were cloned in the pAGGS-IRES-GFP vector and transiently transfected in HEK-293 cells using Trans-IT-293 reagents (Mirus, Madison, MI, USA). Transfected cells were identified by the expression of GFP (green fluorescent protein). Calcium imaging Calcium-imaging experiments were conducted with the fluorescent indicator Fura-2. Cells were incubated with 5 μM Fura-2-acetoxymethylester (Invitrogen) for 60 min at 37 °C. Fluorescence measurements were made with a Zeiss Axioskop FS (Germany) upright microscope fitted with an ORCA ER charge-coupled device camera (Hamamatsu, Japan). Fura-2 was excited at 340 and 380 nm with a rapid switching monochromator (TILL Photonics, Germany). Mean fluorescence intensity ratios (F340/F380) were displayed online with Metafluor software (Molecular Devices, Sunnyvale, USA). The control bath solution contained (in mM) 140 NaCl, 3 KCl, 2.4 CaCl 2 , 1.3 MgCl 2 , 10 HEPES and 10 glucose, and was adjusted to a pH of 7.4 with NaOH. Bath temperature was maintained at 34–36 °C by a custom-built Peltier device. Patch-clamp electrophysiology Whole-cell voltage-clamp recordings were performed with standard patch pipettes (3–6 MΩ resistance) made of borosilicate glass capillaries (Harvard Apparatus Ltd, UK) and contained (in mM) 140 NaCl, 5 CsCl, 10 EGTA, 10 HEPES, (305 mOsm kg −1 ; pH 7.4, adjusted with NaOH). The control bath solution was kept at room temperature except for HC-030031 experiments (32±1 °C). During calcium-free experiments, the bath solution was as follows (in mM): 140 NaCl, 3 KCl, 1.3 MgCl 2 , 10 HEPES, 1 EGTA, 10 glucose. Current signals were recorded with an Axopatch 200B patch-clamp amplifier (Molecular Devices). Stimulus delivery and data acquisition were performed using pClamp 9 software (Molecular Devices). Current development was monitored with repetitive (0.5 Hz) injections of 500 ms duration voltage ramps from −100 to +100 mV, and the voltage steps consisted in a series of 400 ms duration steps ranging from −150 to +175 mV followed by an invariant pulse to −75 mV (400 ms). The holding potential was set to 0 mV. Outside-out patch recordings on mTRPA1 cells were performed in the absence of intracellular and extracellular Ca 2+ . Patch pipettes (3–6 MΩ resistance) contained the standard internal solution (see above) and the calcium-free bath solution (see above). Currents were sampled at 20 kHz and low-pass filtered at 2 kHz. Current development was continuously monitored with repetitive (0.5 Hz) injections of 500 ms duration voltage ramps from −100 to +100 mV from a holding potential of 0 mV. Patch-clamp data were analysed with WinASCD software written by Dr Guy Droogmans ( ftp://ftp.cc.kuleuven.ac.be/pub/droogmans/winascd.zip ) and Origin 7.0 (OriginLab Corporation). Current-clamp recordings of cultured nodose neurons Perforated-patch current-clamp recordings were performed on cultured nodose neurons from adult mice. Standard patch pipettes (2–5 MΩ) were made of borosilicate glass capillaries (Harvard Apparatus Ltd) and contained (in mM) 105 K gluconate, 35 KCl, 10 NaCl, 10 HEPES, 0.1 EGTA and 1 mg ml −1 amphotericin B, pH 7.4. The external solution was identical to the one used in voltage-clamp recordings. Before electrical recordings, neurons expressing TRPA1 were identified with Ca 2+ microfluorimetry (see above) by their response to 10 μM nifedipine, a potent, reversible and non-electrophilic activator of TRPA1 channels [22] . Recordings of lingual nerve afferents The animals were killed by exposure to CO 2 and quickly decapitated. The tongue was carefully dissected, split at the midline and placed in a recording chamber and continuously perfused (3 ml min −1 ) with physiological saline (in mM): NaCl 128, KCl 5, NaH 2 PO 4 1, NaHCO 3 26, CaCl 2 2.4, MgCl 2 1.3 and glucose 10. This solution was gassed with carbogen to pH 7.4. Temperature of the solution was kept around 34 °C and could be modified with a water-cooled, home-designed, Peltier device. Fine filaments of the lingual nerve were split with fine forceps and placed on a platinum electrode for extracellular recording. Electrical signals were alternating current-amplified and high pass filtered. Data were captured and analysed using a CED 1401 interface and Spike 2 software (Cambridge Electronic Design, Cambridge, UK). Single units were detected online using a threshold-based criterion and sorted manually afterwards to remove artefacts. Arterial pressure myography Mice were killed by CO 2 inhalation and decapitation. The mesenteric bed was removed and transferred to ice-cold solution (in mM): NaCl 124, NaHCO 3 25, KCl 5.5, KH 2 PO 4 1.2, MgSO 4 1.2, glucose 5.5, CaCl 2 2.5 (pH 7.4 when aerated with 95% O 2 –5% CO 2 ). Second- and third-branch arteries were removed, dissected free of the adherent fat, cannulated and mounted in a pressure myograph (Danish Myotechnology, Aarhus, Denmark) for measurement of diameter. Before testing the effect of LPS or HC-030031 on arterial tone, arteries were allowed to equilibrate at 70 mm Hg and 37 °C, and after 60 min were precontracted with phenylephrine 2 μM. Assay of TLR4 activity Activation of TLR4 by different forms of ultrapure LPS was tested in HEK-Blue-hTLR4 cells (InvivoGen, San Diego, USA). These HEK-293 cells stably express human TLR4, MD-2, CD14 and an NF-κB-inducible alkaline phosphatase reporter gene system. Expression of secreted alkaline phosphatase was detected with Quanti-Blue (InvivoGen) and quantified by reading the absorbance with a spectrophotometer at 620–655 nm. Cells were maintained in complete DMEM with selective antibiotics, as described by the manufacturer’s instructions (InvivoGen). For testing, cells were plated on 96-well plates at 25,000 cells per well, and were incubated with different concentrations of LPS for 16 h. Analysis of IL-6 levels WT and TRPA1 KO mice were injected i.p. with 0.75 or 1 mg kg −1 E. coli LPS 055:B5 (Sigma-Aldrich) or saline and killed by decapitation 1 h later. Serum and liver were quickly collected and immediately frozen and stored at −80 °C. IL-6 serum levels were determined by enzyme-linked immunosorbent assay (R&D Systems, Minneapolis, USA). Liver analysis of IL-6 messenger RNA levels was performed by reverse transcriptase PCR. Total RNA was extracted using Trizol Reagent (Invitrogen). Reverse transcriptase PCR was performed with a specific set of primers: forward: 5′-GCCACTCCTTCTGTGACTCCAGCT-3′. Reverse: 5′-ACCACTTCACAAGTCGGAGGCTT-3′. Hypoxanthine guanine phosphoribosyl-transferase was used as a housekeeping gene. The amplified products were resolved in a 2% agarose gel and quantified by densitometry using a digital imaging system (Molecular Analyst, Bio-Rad). The PCR products were digested with specific restriction enzymes to determine their specificity. CGRP enzyme immunoassay and analysis The CGRP content of the incubation fluid was measured using a commercial enzyme immunoassay kits with a detection threshold of 2 pg ml −1 (Bertin Pharma, Montigny-le-Bretonneux, France). For this purpose, 100 μl fluid samples were stored on ice and mixed, immediately following the trachea incubation period, with 25 μl of fivefold concentrated commercial CGRP enzyme immunoassay buffer that contained a cocktail of peptidase inhibitors. The CGRP contents were determined after the end of the experiment; the antibody reactions took place overnight. Enzyme immunoassay plates were scored photometrically using a microplate reader (Dynatech, UK). All results are presented as measured by the enzyme immunoassay in pg CGRP per ml incubation fluid. To reduce interindividual and day-to-day baseline variability, the data were normalized to the second baseline value (before any stimulation). This value was subtracted from all data points so that only the absolute change in CGRP release (Δ pg ml −1 ) is displayed in the figures. Statistical comparisons were performed using the Statistica 7 software (Statsoft, Tulsa, USA). The baseline-normalized ΔCGRP values were entered into a one-way analysis of variance followed by Fisher’s least significant difference test, focusing on the peak values of stimulated CGRP release; * P <0.05 was considered significant. Data points represent means±s.e.m. of the given number ( n ) of experiments. Behavioural testing Behavioural studies were performed on littermates that were wild type or homozygous null at the Trpa1 or Tlr4 allele. All experiments were scored by a tester blind to genotype and to drugs injected. A total of 51 wild type, 25 Trpa1 KO and 6 Tlr4 KO male mice (2–3 months old) were used. To measure acute nocifensive responses, mice were placed within transparent plastic cylinders and allowed to accommodate for 2 h. LPS (5 μg μl −1 ) was prepared in PBS and delivered via intraplantar injection in a volume of 10 μl using a 30 G needle coupled to a Hamilton syringe. Immediately after injection, nocifensive time was scored as the total time spent licking, lifting, guarding, shaking or biting of the injected hind paw over a period of 10 min. A separate group of animals received injection of vehicle alone. Mechanical thresholds were determined with Von Frey hairs using a modified version of Dixon’s up-down method [67] . Procedures and intraplantar dosis of LPS were identical to those used for nocifensive responses. Mice were placed in transparent plastic cylinders (13 cm diameter × 8 cm height) on a metal mesh platform and calibrated von Frey filaments were applied to the plantar surface of the hind paw for up to 2 s with sufficient force to cause the filament to bow. Brisk withdrawal of the hind paw during or immediately after application was considered a positive response. The threshold force required to elicit withdrawal of the paw (50% hind paw withdrawal) was determined from two separate trials. Data presented are from both left and right hind paws averaged together, as there were no laterality effects. To examine the effects of LPS on body temperature (Tb), animals (adult male mice) were adapted to a Plexiglass chamber (15 × 15 × 30 cm 3 ) in a room at 23±1 °C. Baseline rectal temperature was recorded with a thermoprobe connected to a digital thermometer (Lendhermack, model IM902C). At time zero (10:00 day time), immediately after a second measure of Tb, vehicle (PBS) or 3 mg kg −1 of E. coli LPS were injected i.p. Thereafter, Tb was monitored at 1 h interval for 7 h, and the following morning. Chemical reagents LPS from E. coli , S. typhimurium, S. minnesota and P. aeruginosa (purified by gel-filtration chromatography), and K. pneumoniae , S. marcescens (purified by phenol extraction) were purchased from Sigma-Aldrich. N. meningitidis LPS was purified by phenol extraction at the Center for Vaccines Research and Production (Finlay Institute, Havana, Cuba). The quality of this LPS (40.5 × 10 6 EU ml −1 ) was determined with a Kinetic-QCL Limulus amebocyte lysate, using the programme Wiea QCL and a Lonza kit. LPSs were dissolved as a stock solution in endotoxin-free distilled water, or PBS for behavioural experiments, at a concentration of 5 mg ml −1 . Other ultrapure forms of LPS were purchased from InvivoGen (San Diego, USA), obtained by repeated phenol extractions and prepared as sterile stock solutions with sterile water and diluted right before use. These included LPS from E. coli strain 0111:B4, S. minnesota and R. sphaeroides . Table 1 summarizes the source and characteristics of the different LPS used. Table 1 List of LPS reagents used in the study, purity and supplier . Full size table Diphosphoryl lipid A (from E. coli F583 Rd mutant, Sigma) was dissolved in a glass tube at a concentration of 1 mg ml −1 in chloroform/methanol (3:1 v/v). The suspension was heated up to 40 °C and solvent was dried by rotary evaporation under a stream of N 2 . The glass tubes were supplemented with extracellular solution and subjected to sonication for 40 min. Synthetic monophosphoryl lipid A (InvivoGen) was prepared as a 1-mg ml −1 solution in dimethyl sulphoxide (DMSO). Control experiments contained the same concentration of vehicle. CLI-095 (InvivoGen), also known as TAK-242, was prepared as a 3-mM stock solution in DMSO. Polymyxin B (InvivoGen) was prepared as a 50-mg ml −1 stock in distilled water. AITC, CA, TNP and HNE were stored as stock solutions and diluted immediately before the experiments. HC-030031 was purchased from Tocris and stored in a DMSO solution at 100 mM. Data analysis Data are reported as mean±s.e.m. Dose–response data were normalized to the maximum response of the drug in each case and then were fitted with the Hill equation using the Levenberg–Marquardt method implemented in Origin 7.0 software. The s.e.m. were used as weights in fitting where applicable. When comparing two means, statistical significance ( P <0.05) was assessed by Student’s two-tailed t -test. When comparing proportions between two experimental groups (for example, percentage of responding neurons), we used Fisher’s exact test. How to cite this article: Meseguer, V. et al . TRPA1 channels mediate acute neurogenic inflammation and pain produced by bacterial endotoxins. Nat. Commun. 5:3125 doi: 10.1038/ncomms4125 (2014).